Selective suppression of excessive GluN2C expression rescues early epilepsy in a tuberous sclerosis murine model Tuberous sclerosis complex (TSC), caused by dominant mutations in either TSC1 or TSC2 tumour suppressor genes is characterized by the presence of brain malformations, the cortical tubers that are thought to contribute to the generation of pharmacoresistant epilepsy. Here we report that tuberless heterozygote Tsc1 +/− mice show functional upregulation of cortical GluN2C-containing N-methyl-D-aspartate receptors (NMDARs) in an mTOR-dependent manner and exhibit recurrent, unprovoked seizures during early postnatal life (<P19). Seizures are generated intracortically in the granular layer of the neocortex. Slow kinetics of aberrant GluN2C-mediated currents in spiny stellate cells promotes excessive temporal integration of persistent NMDAR-mediated recurrent excitation and seizure generation. Accordingly, specific GluN2C/D antagonists block seizures in Tsc1 +/− mice in vivo and in vitro . Likewise, GluN2C expression is upregulated in TSC human surgical resections, and a GluN2C/D antagonist reduces paroxysmal hyperexcitability. Thus, GluN2C receptor constitutes a promising molecular target to treat epilepsy in TSC patients. Tuberous sclerosis complex (TSC) is an autosomal-dominant disease affecting multiple organ systems (brain, skin, kidney, heart and lung) and caused by germline mutations in one of the tumour suppressor genes, TSC1 or TSC2 (ref. 1 ). Inactivation of either of these genes leads to hyperactivation of the mammalian target of rapamycin (mTOR) pathway and promotes neuropathological abnormalities associated with TSC [2] , [3] , [4] . The most devastating clinical and pathological expressions of TSC involves the central nervous system, and includes malformative brain lesions, the cortical tubers, epilepsy, autism, cognitive impairment and glial tumours [5] . Epilepsy begins in infancy and is difficult to treat with 85–90% patients remaining with pharmacoresistant seizures [5] . The molecular mechanisms governing epileptogenesis in TSC and the contribution of tuber formation have been intensively studied during the last decade and were subjects of intensive debates. Recent evidence indicates that gliomas are formed by biallelic TSC1 or TSC2 gene inactivation, reflecting a double-hit mechanism according to which a germline or a somatic mutation (likely occurring during development) affects the non-mutated allele, producing ‘loss of heterozygosity’ [6] . However, loss of heterozygosity at either TSC gene is a rare event in tubers in human [7] , and although it may affect selected population of giant cells within cortical tubers, most of the cells in whole tuber sections have heterozygote mutations [8] . Although correlations have been found between severity of the condition and the number of tubers [9] , [10] , and between topography of cortical tubers and type of epilepsy, it remains elusive whether tubers are intrinsically epileptogenic as some patients with numerous tubers have a benign condition, whereas some others, without tubers, have extremely severe epilepsy [11] , [12] , [13] , [14] . Furthermore, the epileptogenic zone may not be exactly superimposed to the lesion and includes some adjacent or, more rarely, remote areas [12] . This could explain why for approximately one-third of individuals who undergo epilepsy surgery, seizures persist after removal of the cortical tubers suspected to be epileptogenic [9] , [10] . Thus, it is not clear what mechanisms underlie epilepsy in perituberal region and in patients without evidence of cortical tubers or other dysgenetic features. Numerous animal models of TSC have been generated in order to evaluate the mechanisms by which TSC genes loss results in the diverse pathological phenotypes. Mouse models generated using different brain-specific promoters and conditional alleles, in which both alleles of either Tsc1 or Tsc2 are lost in neurons or glia, display a severe neurological phenotype including morphological and clinical TSC features such as tuber-like structures, failure to thrive, frequent seizures and early mortality [15] , [16] , [17] , [18] . However, both heterozygous Tsc1 and Tsc2 knockout mice demonstrate behavioural and electrophysiological abnormalities and cognitive dysfunction in the absence of tubers or seizures [4] , [19] , [20] . This supports the concept that haploinsufficiency of Tsc1 or Tsc2 expression contributes significantly to the brain manifestations of TSC, although epileptic phenotype has not been reported so far for these mice. Possible mechanisms of seizure generation in TSC could include changes in excitatory and inhibitory neurotransmitter function that may lead to abnormal neuronal synchronization and imbalance between excitation and inhibition [21] , [22] . Several reports have shown an increased expression of excitatory amino-acid binding sites in the epileptic cortex and altered ionotropic glutamate receptors expression patterns in human cortical tubers [23] , [24] , [25] , [26] . N -methyl- D -aspartate receptors (NMDARs) are putative candidates to explain the hyperexcitability of TSC neuronal networks. Slow decay kinetics of the currents mediated by NMDARs could facilitate synchronization in neuronal networks and thus exert proepileptic effects. However, the functional and proepileptic significance of NMDARs in epileptogenesis associated with TSC has not been explored. In this study, we report that heterozygote Tsc1 +/− mice show functional upregulation of cortical GluN2C-containing NMDARs and exhibit spontaneous seizures associated with clinical manifestations during early postnatal life (<P19) despite the absence of major morphological changes in the brain [15] , [20] . Selective inhibition of these receptors strongly disrupts spontaneous epileptiform activity in Tsc1 +/− mice. Furthermore, electrophysiological and quantitative real-time reverse transcription polymerase chain reaction (RT-PCR) analysis of postsurgical tissue from TSC patients reveal upregulation of GluN2C subunits, indicating that these NMDAR subunits are instrumental in human TSC. Collectively, these observations suggest that an upregulation of GluN2C subunits is of paramount importance in the manifestation of epileptic phenotypes associated with TSC. Spontaneous seizures in Tsc1 +/− mice To characterize functional abnormalities of haploinsufficient Tsc1 +/− mice, lacking major malformations [15] , [20] , in vivo intracortical electroencephalography (EEG) recordings in somatosensory S1 cortex of head-restrained non-anaesthetized Tsc1 +/− mice at postnatal days P9–P33 were performed. Spontaneous recurrent seizures occurred in 77% of Tsc1 +/− mice tested at P9–P18 (26 out of 34), but were not observed in Tsc1 wt mice of the same age ( Fig. 1 and Supplementary Figs 1 and 2 ). The seizures started 2–3 h after onset of EEG recordings and recurred as often as six per hour. Ictal discharges were often associated with screaming, oro-facial automatisms, head tremor, straub tail and tonic-clonic seizures ( Supplementary Movie 1 ), followed by a quiet behaviour ( Supplementary Movie 2 ). 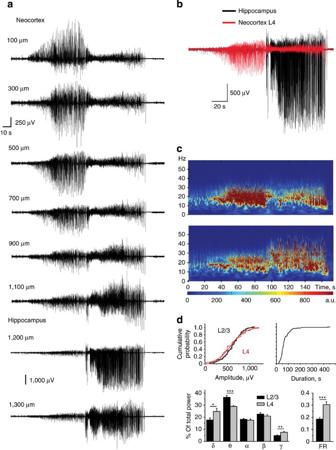Figure 1: Spontaneous seizures inTsc1+/−mice. (a) Intracortical EEG recorded using a 16-channel silicone probe in a head-restrained P16Tsc1+/−mouse. The upper channel corresponds to the superficial intracortical electrode placed at 100 μm from the pia. Shown are epileptic discharges recorded at the depths indicated on the left of each trace. (b) Superimposed epileptic discharges in L4 of neocortex (red) and hippocampus (black). (c) Wavelet analysis during the ictal events for traces shown inb. Upper panel: neocortex, lower panel: hippocampus. (d) Cumulative probabilities of seizures maximal amplitudes for L2/3 and L4 (upper left,n=84 seizures,N=20 mice) and durations (upper right,n=104 seizures,N=20). Seizure durations were the same for all layers, data for L2/3 are shown. Bottom: relative integral power of δ-(1–4 Hz), θ-(4–8 Hz), α-(8–12 Hz), β-(12–25 Hz), γ-(25–100 Hz) and fast ripple (FR; 100–500 Hz) band components of EEG in L2/3 (n=31 seizures,N=20) and L4 (n=29 seizures,N=20) revealed by Fourier transform analysis. All means±s.e.m.; *P<0.05, **P<0.01, ***P<0.001, two-sample two-tailedt-test. Figure 1: Spontaneous seizures in Tsc1 +/− mice. ( a ) Intracortical EEG recorded using a 16-channel silicone probe in a head-restrained P16 Tsc1 +/− mouse. The upper channel corresponds to the superficial intracortical electrode placed at 100 μm from the pia. Shown are epileptic discharges recorded at the depths indicated on the left of each trace. ( b ) Superimposed epileptic discharges in L4 of neocortex (red) and hippocampus (black). ( c ) Wavelet analysis during the ictal events for traces shown in b . Upper panel: neocortex, lower panel: hippocampus. ( d ) Cumulative probabilities of seizures maximal amplitudes for L2/3 and L4 (upper left, n =84 seizures, N =20 mice) and durations (upper right, n =104 seizures, N =20). Seizure durations were the same for all layers, data for L2/3 are shown. Bottom: relative integral power of δ-(1–4 Hz), θ-(4–8 Hz), α-(8–12 Hz), β-(12–25 Hz), γ-(25–100 Hz) and fast ripple (FR; 100–500 Hz) band components of EEG in L2/3 ( n =31 seizures, N =20) and L4 ( n =29 seizures, N =20) revealed by Fourier transform analysis. All means±s.e.m. ; * P <0.05, ** P <0.01, *** P <0.001, two-sample two-tailed t -test. Full size image Ictal EEG patterns started as high-frequency, low-amplitude activity that progressively evolved to high-amplitude regular polyspike trains involving all cortical layers. Subsequently, there were disruptions of the discharges with a reduction in EEG amplitude in cortex and appearance of high-amplitude rhythmic spike-wave trains in the hippocampus ( Fig. 1a,b ). Wavelet analysis showed an increase in high-frequency activity during ictal discharges ( Fig. 1c ). The contributions of δ, γ and fast ripple bands in power spectrum during discharges were significantly larger in neocortical layer 4 (L4) compared with layer 2/3 (L2/3; Fig. 1d , bottom panels). The amplitude and duration of discharges varied within litters with a mean amplitude of 615±18 μV and a mean duration of 70.3±5 s, ( n =104 seizures; N =20 mice; Fig. 1d , upper panels). Interestingly, epileptic phenotype was not observed in Tsc1 +/− mice at ages older than P19 (P19–P33, N =10), indicating that this is a developmental insult. The seizure onset as well as the peaks of averaged population spikes in L4 preceded those in L2/3 ( Supplementary Fig. 3a , mean delay for the peaks was 8.0±1.3 ms, N =11 mice). These observations and current source density (CSD) analysis suggest that epileptic activities in the cortex are initiated in granular cortical layer before spreading to supra- and infragranular layers ( Supplementary Fig. 3b ). Qualitatively, similar results were obtained in coronal slices of Tsc1 +/− mouse brains, where intralaminar circuitry and horizontal recurrent connections were intact, but thalamo–cortical inputs were absent. In simultaneous whole-cell recordings from somatosensory cortical excitatory neurons in L4 and L2/3 spontaneous synchronized bursts were observed first in L4 and subsequently in L2/3 neurons with an average delay of 30.4±5.5 ms (61 synchronous bursts were analysed; Fig. 2a,b ). Therefore, L4 neurons have a central role in neocortical epileptogenesis in Tsc1 +/− mice. 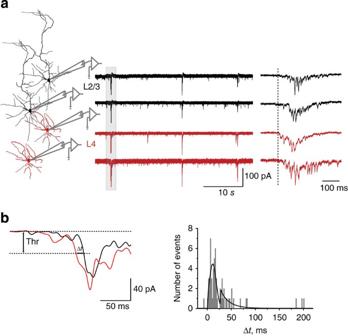Figure 2: Onset of spontaneous synchronous bursts in L4 preceded that in L2/3. (a) Middle: traces of whole-cell currents recorded atVh=−70 mV simultaneously from two PNs in L2/3 and two SSCs in L4 (shown schematically on the left) in neocortical slices fromTsc1+/−mice. Right: expanded traces of the same bursts marked by grey box are shown. Vertical dotted line outlines bursts onset in L4. Note that onsets of the bursts in L4 precede those in L2/3. (b) Distribution of the onset delays (Δt) between bursts recorded simultaneously from L2/3 and L4 neurons (61 synchronous bursts were analysed,N=4 mice). Δtwas measured from filtered (0.5 kHz) events at the level of the burst threshold (Thr) set at 40 pA as shown on the left. Events with amplitude <40 pA were not considered as the bursts. Fitting a Gaussian Function of Δtdistribution revealed at least two peaks with the most of the Δtvalues peaking at 12 ms. Figure 2: Onset of spontaneous synchronous bursts in L4 preceded that in L2/3. ( a ) Middle: traces of whole-cell currents recorded at V h =−70 mV simultaneously from two PNs in L2/3 and two SSCs in L4 (shown schematically on the left) in neocortical slices from Tsc1 +/− mice. Right: expanded traces of the same bursts marked by grey box are shown. Vertical dotted line outlines bursts onset in L4. Note that onsets of the bursts in L4 precede those in L2/3. ( b ) Distribution of the onset delays (Δ t ) between bursts recorded simultaneously from L2/3 and L4 neurons (61 synchronous bursts were analysed, N =4 mice). Δ t was measured from filtered (0.5 kHz) events at the level of the burst threshold (Thr) set at 40 pA as shown on the left. Events with amplitude <40 pA were not considered as the bursts. Fitting a Gaussian Function of Δ t distribution revealed at least two peaks with the most of the Δ t values peaking at 12 ms. Full size image Upregulation of GluN2B and GluN2C/D NMDARs in Tsc1 +/− mice L4 is the main collector of sensory information and cortical ‘hub’ for intracolumnal information processing [27] . Recurrent activity triggered within the highly interconnected networks of L4 has been suggested to act to selectively amplify and redistribute transient high-frequency thalamo–cortical inputs [28] , [29] . What are the mechanisms underlying the increased integrative capacity of L4 neurons in Tsc1 +/− mice? As NMDARs have an important role in L4 neuron integrative properties [30] , [31] , we next examined whether slow NMDAR-mediated signalling was altered in Tsc1 +/− mice. The L4–L4 connections are almost the only intracortical synaptic input that L4 spiny stellate cells (SSCs) receive [32] . This allows an estimation of the contribution of the slow NMDA component in isolated L4–L4 connections by measuring spontaneous activity from SSCs. To monitor the NMDAR-mediated current, we performed whole-cell recordings of spontaneous excitatory postsynaptic currents (sEPSCs) from L4 SSCs ( Fig. 3a ) and L2/3 pyramidal neurons (PNs) in coronal brain slices from Tsc1 +/− mice (P14–P16) in voltage-clamp mode at −50 mV. The decay kinetics of the composite sEPSCs was significantly slower in Tsc1 +/− than that in Tsc1 wt mice both in L2/3 and L4 neurons ( Fig. 3b,c ), suggesting an increased contribution of NMDAR-mediated current and an upregulation of GluN2B, and/or GluN2C and GluN2D NMDAR subunits endowed with slow decay kinetics [33] . To quantify alterations in sEPSCs decay, we measured charge transfer normalized by the peak amplitude (see Methods section for details). In Tsc1 +/− mice, normalized charges of sEPSC were 1.5±0.1 in L2/3 and 2.55±0.16 in L4 of those in Tsc1 wt mice (L2/3: n =27 and 16 neurons; L4: n =34 and 29 neurons for Tsc1 +/− and Tsc1 wt mice, respectively; two-sample, two-tailed t -test Tsc1 wt versus Tsc1 +/− in L2/3 P <5 × 10 − 4 , and in L4 P <1 × 10 − 11 ). Bi-exponential-weighted time constants of sEPSC decay ( τ w ) were in Tsc1 wt mice 7.5±0.6 ms for L2/3 and 7.4±0.4 ms for L4, and in Tsc1 +/− mice 13.28±0.97 ms for L2/3 and 16.76±1.19 ms for L4 (two-sample, two-tailed t -test Tsc1 wt versus Tsc1 +/− in L2/3 P <2 × 10 − 4 , and in L4 P <8 × 10 − 9 ). Corresponding amplitudes of sEPSC in Tsc1 +/− mice were not significantly different from those in Tsc1 wt mice in L4 (two-sample, two-tailed t -test, P >0.7), however, they were slightly increased in L2/3 (two-sample, two-tailed t -test, P <0.07; Supplementary Fig. 4 ). 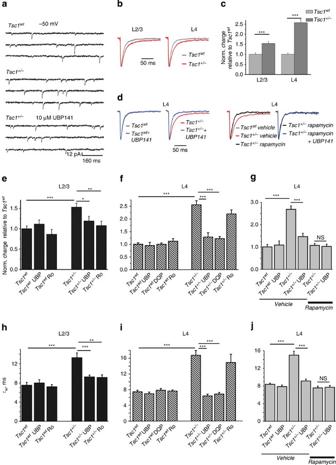Figure 3: Layer-specific functional upregulation of GluN2B and GluN2C/D subunits containing NMDA receptors inTsc1+/−mice. (a) Representative traces of spontaneous activity recorded in whole-cell mode at holding potential −50 mV from SSCs in L4 in neocortical coronal slices fromTsc1wt,Tsc1+/−mice and inTsc1+/−mice in the presence of UBP141 (10 μM). (b) Grand averages of normalized (Norm.) and superimposed traces of sEPSC recorded from PNs in L2/3 (left) or SSCs in L4 (right) inTsc1wtandTsc1+/−mice at −50 mV. For each neuron, original traces from individual experiments were aligned based on the starts of their rising phases and averaged. These averaged traces from individual experiments were normalized and averaged to form grand average traces shown. Pooled data from 16 neurons forTsc1wt(N=5 mice) and 27 neurons forTsc1+/−in L2/3 (N=8) and from 29 neurons forTsc1wt(N=6) and 34 neurons forTsc1+/−in L4 (N=10). (c) Summary data for normalized charges of sEPSC in L2/3 and L4 inTsc1wtand inTsc1+/−mice (relative toTsc1wt). (d) Left two panels: superimposed grand average of normalized traces of sEPSC recorded in L4 inTsc1wtandTsc1+/−mice in control and in the presence of UBP141. Right two panels: superimposed grand average of normalized traces of sEPSC recorded in L4 inTsc1+/−andTsc1wtmice pretreated with either vehicle or rapamycin. (e,h) Summary data for the effects of UBP141 and Ro25-6981 (1 μM) on normalized charges of sEPSC (e) and weighted time constant,τw(h) of sEPSC decay in L2/3 inTsc1wtand inTsc1+/−mice. (f,i) Summary data for the effects of UBP141, DQP1105 (10 μM) and Ro25-6981 on normalized charges of sEPSC (f) andτw(i) in L4 inTsc1wtand inTsc1+/−mice. (g,j) Summary data for the effects of UBP141 on normalized charges of sEPSC (g) andτW(j) in L4 inTsc1wtand inTsc1+/−mice pretreated with either vehicle or rapamycin. All means±s.e.m. All data sets were analysed using one-way ANOVA followed by Fisher’s Least Significant Difference (LSD)post hoctest (seeSupplementary Table 2for statistics); *P<0.05, **P<0.01, ***P<0.001. NS, not significant,. Figure 3: Layer-specific functional upregulation of GluN2B and GluN2C/D subunits containing NMDA receptors in Tsc1 +/− mice. ( a ) Representative traces of spontaneous activity recorded in whole-cell mode at holding potential −50 mV from SSCs in L4 in neocortical coronal slices from Tsc1 wt , Tsc1 +/− mice and in Tsc1 +/− mice in the presence of UBP141 (10 μM). ( b ) Grand averages of normalized (Norm.) and superimposed traces of sEPSC recorded from PNs in L2/3 (left) or SSCs in L4 (right) in Tsc1 wt and Tsc1 +/− mice at −50 mV. For each neuron, original traces from individual experiments were aligned based on the starts of their rising phases and averaged. These averaged traces from individual experiments were normalized and averaged to form grand average traces shown. Pooled data from 16 neurons for Tsc1 wt ( N =5 mice) and 27 neurons for Tsc1 +/− in L2/3 ( N =8) and from 29 neurons for Tsc1 wt ( N =6) and 34 neurons for Tsc1 +/− in L4 ( N =10). ( c ) Summary data for normalized charges of sEPSC in L2/3 and L4 in Tsc1 wt and in Tsc1 +/− mice (relative to Tsc1 wt ). ( d ) Left two panels: superimposed grand average of normalized traces of sEPSC recorded in L4 in Tsc1 wt and Tsc1 +/− mice in control and in the presence of UBP141. Right two panels: superimposed grand average of normalized traces of sEPSC recorded in L4 in Tsc1 +/− and Tsc1 wt mice pretreated with either vehicle or rapamycin. ( e , h ) Summary data for the effects of UBP141 and Ro25-6981 (1 μM) on normalized charges of sEPSC ( e ) and weighted time constant, τ w ( h ) of sEPSC decay in L2/3 in Tsc1 wt and in Tsc1 +/− mice. ( f , i ) Summary data for the effects of UBP141, DQP1105 (10 μM) and Ro25-6981 on normalized charges of sEPSC ( f ) and τ w ( i ) in L4 in Tsc1 wt and in Tsc1 +/− mice. ( g , j ) Summary data for the effects of UBP141 on normalized charges of sEPSC ( g ) and τ W ( j ) in L4 in Tsc1 wt and in Tsc1 +/− mice pretreated with either vehicle or rapamycin. All means±s.e.m. All data sets were analysed using one-way ANOVA followed by Fisher’s Least Significant Difference (LSD) post hoc test (see Supplementary Table 2 for statistics); * P <0.05, ** P <0.01, *** P <0.001. NS, not significant,. Full size image To directly determine the involvement of NMDAR subtypes in prolongation of sEPSCs, we used specific GluN2B (Ro25-6981) and GluN2C/D (UBP141 (ref. 34 ), and DQP1105 (ref. 35 )) antagonists ( Supplementary Table 1 ). In L4 SSCs in Tsc1 +/− mice UBP141 and DQP1105, but not Ro25-6981, accelerated sEPSCs decay, restoring it to the values in Tsc1 wt mice ( Fig. 3d,f,i and Supplementary Table 2 ), suggesting an increased contribution of GluN2C/D but not GluN2B subunits. In Tsc1 +/− mice, the normalized charge of sEPSC in L4 in the presence of UBP141 (10 μM) was 0.61±0.07 ( n =10, P <4 × 10 − 4 , paired two-tailed t -test) and in the presence of DQP1105 (10 μM) was 0.48±0.04 ( n =12, P <2 × 10 − 7 , paired two-tailed t -test) of that without drugs. Relative τ w values were 0.56±0.06 for UBP141 ( P <5 × 10 − 5 , paired two-tailed t -test) and 0.41±0.04 for DQP1105 ( P <3 × 10 − 8 , paired two-tailed t -test), respectively, of those without drugs. In Tsc1 wt mice, sEPSCs decay kinetics was not affected by either drug (the normalized charge values were similar in the presence and absence of the drugs: 1.03±0.13, n =9, P >0.75 for UBP141 and 1.06±0.07, n =12, P >0.4 for DQP1105; paired two-tailed t -test). Correspondingly, the relative τ w values were 0.98±0.07, P >0.3 for UBP141 and 1.07±0.07, P >0.7 for DQP1105 (paired two-tailed t -test). Corresponding amplitudes of sEPSC for all sets were not significantly different (analysis of variance (ANOVA), P >0.9; Supplementary Fig. 4 ). In addition, we performed recordings of miniature EPSCs (mEPSCs) in L4 cells in the presence of tetrodotoxin (1 μM). Similarly to sEPSCs, the average decay kinetics of the late component in composite mEPSCs was significantly slower in Tsc1 +/− than that in Tsc1 wt mice ( Supplementary Fig. 5 ). Thus, in Tsc1 +/− mice, averaged normalized charge of mEPSC in L4 was 2.58±0.18 of that in Tsc1 wt mice ( n =10 and 9 neurons, for Tsc1 +/− and Tsc1 wt mice, respectively; two-sample, two-tailed t -test Tsc1 wt versus Tsc1 +/− P <5 × 10 − 7 ). In Tsc1 +/− mice, the normalized charge of mEPSC and τ w in L4 in the presence of DQP1105 (10 μM) were 0.45±0.07 ( n =8, P <1.7 × 10 − 4 , paired two-tailed t -test) and 0.55±0.03 ( n =9, P <3.2 × 10 − 5 , paired two-tailed t -test), respectively of those without drugs. In Tsc1 wt mice, mEPSCs decay kinetics were not affected by DQP1105: the normalized charge and τ w in the presence of DQP1105 were 0.96±0.14 ( n =7, P >0.75, paired two-tailed t -test) and 1.13±0.13 ( n =8, P >0.48, paired two-tailed t -test), respectively, of those without drug. Corresponding amplitudes of mEPSC for all sets were not significantly different (ANOVA, P >0.9; Supplementary Fig. 5 ). In contrast to the data in L4, the contribution of both GluN2B and GluN2C/D subunits was increased in L2/3 of Tsc1 +/ − mice. Both Ro25-6981 and UBP141 accelerated sEPSC decay ( Fig. 3e,h ). In the presence of 1 μM Ro25-6981, the normalized sEPSC charge in Tsc1 +/− mice was 0.79±0.05 of control without Ro25-6981 ( n =9, P <0.005, paired two-tailed t -test). In Tsc1 wt mice, this value was 1.03±0.09 ( n =6, P >0.75, paired two-tailed t -test). Similarly, corresponding numbers for UBP141 in L2/3 were 0.8±0.07 of controls without the drug ( n =12, P <0.02, paired two-tailed t -test) in Tsc1 +/ − mice and 1.02±0.07 ( n =9, P >0.8, paired two-tailed t -test) in Tsc1 wt mice. However, the interpretation of UBP141 effects in L2/3 is complicated by the fact that at a concentration of 10 μM it partially affects also GluN2B receptors ( Supplementary Table 1 ). The amplitudes of sEPSCs in the presence of antagonists were not significantly different from control values for all experimental sets (ANOVA, P >0.15; Supplementary Fig. 4 ). Therefore, there is an increased contribution of GluN2C/D subunits in L4, but of both GluN2B and GluN2C/D subunits in L2/3 in Tsc1 +/ − mice when compared with naive Tsc1 wt mice. To determine whether upregulation of the GluN2C/D-NMDAR component in L4 is a direct consequence of enhanced mTOR signalling caused by Tsc1 inactivation, we performed experiments in Tsc1 +/− mice chronically treated with the mTOR inhibitor rapamycin (see Methods section). Recordings of sEPSC from SSCs in L4 in rapamycin-treated Tsc1 +/− mice (P14–P16) showed the absence of the UBP141-sensitive component ( Fig. 3d,g,j ). In rapamycin-treated Tsc1 +/− mice, the normalized charge of sEPSCs in SSCs in the presence of UBP141 (10 μM) was 1.05±0.11 ( n =12, P >0,6, paired two-tailed t -test) of that without the drug. Furthermore, normalized charge of sEPSCs in rapamycin-treated Tsc1 +/− mice was not significantly different from that of vehicle-treated Tsc1 wt mice (1.05±0.08 of that in vehicle-treated Tsc1 wt mice, n =14 for Tsc1 +/− , n =10 for Tsc1 wt , two-sample two-tailed t -test P >0.75; Fig. 3g ). This finding indicates a crucial role of mTOR signalling in functional upregulation of GluN2C/D-containing NMDARs in Tsc1 +/− mice. Interestingly, in L4 fast-spiking (FS) interneurons neither UBP141 nor Ro25-6981 altered sEPSCs decay in both Tsc1 wt and Tsc1 +/− mice ( Supplementary Fig. 6 ), suggesting that NMDAR-mediated currents in inhibitory neurons remain intact. To further determine the functional effects of UBP141 in Tsc1 +/− mice, we tested its actions on the amplitude and frequency of α -amino-3-hydroxy-5-methyl-4-isoxazolepropionic acid receptor (AMPAR)-mediated sEPSCs. UBP141 altered neither the amplitude nor the kinetics of AMPAR-mediated sEPCS recorded at −80 mV in L4 SSCs ( Supplementary Fig. 7a,b ). The frequency of sEPSCs recorded at −80 mV in L4 SSCs was not different from that in Tsc1 wt mice. However, in L2/3 PNs it was significantly higher than that of Tsc1 wt mice ( Supplementary Fig. 7c ), and was reduced by bath application of UBP141 in Tsc1 +/− ( Supplementary Fig. 7e ), but not in Tsc1 wt ( Supplementary Fig. 7d ) mice. Therefore, in Tsc1 +/− mice L4 GluN2B/C/D channels presynaptic to L2/3 PN could contribute to increase the activity of the latter. mTOR-dependent upregulation of the slow NMDAR subunits was confirmed by quantitative RT–PCR revealing 2.4-fold elevation of GluN2C mRNAs ( P <0.005, two-tailed t -test) in the neocortex of Tsc1 +/− mice ( N =5) compared with age-matched Tsc1 wt ( N =5) mice ( Supplementary Fig. 8 ). Thus, the contribution of GluN2C-containing NMDARs with slow kinetics is increased in neocortical L4 and L2/3 excitatory neurons in mice with haploinsufficient Tsc1 mutation. Similar alterations in sEPSC kinetics were observed in ‘double-hit’ Tsc1 mutant mice. In a recent study, using in utero electroporation and relying on the «second-hit» mutation concept [36] , Bordey and co-workers [15] generated a Tsc1 −/− animal model with the hallmark of human TSC, namely the tubers. We used this model to test the impact of a «second-hit» mutation on functional upregulation of slow NMDARs. To do that, Tsc1 flx/mut mice (as well as Tsc1 flx/wt ) were injected in utero at embryonic day 16 (E16) with pCAG-mRFP alone or combined with pCAG-Cre:GFP to induce, after electroporation, deletion of the floxed Tsc1 gene in a subset of neurons. The fluorescence of the monomeric red fluorescent protein (mRFP) plasmid allows identification of electroporated neurons and green fluorescent protein (GFP) for detection of neurons containing pCAG-Cre. Whole-cell recordings in neocortical slices from mRFP + /GFP + neurons of Tsc1 flx/mut ; pCAG-Cre and Tsc1 flx/wt ; pCAG-Cre conditional knockout mice (hereafter referred to as Tsc1 null and Tsc1 haplo neurons, respectively) at −50 mV revealed enhanced contribution of slow UBP141-sensitive NMDAR-mediated components in sEPSC compared with those from control mRFP + neurons of Tsc1 flx/wt mice, in the same manner as in non-electroporated heterozygote Tsc1 +/− mice. Therefore, GluN2C/D-mediated currents are present in both Tsc1 haplo and «double-hit» Tsc1 null neurons. Importantly, the extent of slow NMDARs contribution was the same for the electroporated neurons with heterozygote and homozygote Tsc1 mutations ( Supplementary Fig. 9 ). Slow NMDAR-mediated signal determines temporal integration To test temporal summation at γ-band frequency, we performed simultaneous whole-cell recordings from pairs of synaptically coupled SSCs in L4 of somatosensory cortex in slices from Tsc1 +/− and Tsc1 wt P14–P16 mice. The majority of interconnected excitatory neurons were SSCs with an asymmetrical dendritic arborization largely confined to L4 and characteristics action potentials firing pattern ( Fig. 4a,b ). In concordance with the slower NMDAR-mediated component of synaptic transmission in Tsc1 +/− mice, recordings revealed a significantly higher extent of temporal integration compared with Tsc1 wt mice when measuring EPSCs evoked by stimulation of presynaptic cells with a train of action potentials. Normalized charge transfer of the train-EPSCs estimated from normalized by the amplitude of the first peak currents was 0.093±0.004 s in Tsc1 +/− ( n =5) and 0.050±0.006 s ( n =7) in Tsc1 wt mice, respectively, ( P <0.0005, two-tailed t -test; Fig. 4c–e ). Furthermore, recordings in Tsc1 +/− mice demonstrated significantly increased contribution of UBP141-sensitive NMDAR-mediated train-EPSCs to the postsynaptic summation of EPSCs but not in Tsc1 wt mice ( Fig. 4d,f,g ). In the presence of UBP141, the normalized sEPSC charge in Tsc1 +/− mice was 0.57±0.11 of that without UBP141 ( n =4, P <0.03, paired two-tailed t -test). In Tsc1 wt mice, this value was 1.06±0.07 ( n =6, P >0.44, paired two-tailed t -test). Thus, abnormal slowing of the NMDAR-mediated current kinetics increases temporal integration within recurrent network in L4 of Tsc1 +/− mice. 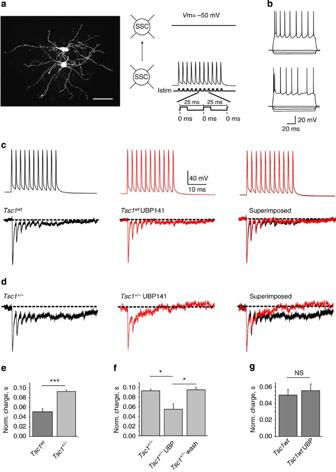Figure 4: Enhanced temporal integration of synaptic responses in synaptically coupled SSCs in L4 inTsc1+/−mice. (a) Fluorescence images from two SSCs (left) and the configuration of a paired recordings (right). Scale bar, 50 μm. (b) Representative action potential firing patterns of both, postsynaptic (top) and presynaptic (bottom) SSCs recorded in current clamp mode. (c,d) Representative averaged normalized by the first peaks in the trains traces of EPSCs recorded in voltage-clamp mode in pairs of SSCs in L4 (averaged 25 sweeps) fromTsc1wt(c, bottom panels) andTsc1+/−(d) mice induced by train stimulation (11 stimuli at 40 Hz) in presynaptic cell in the absence (left panels, black traces) or presence (middle panels, red traces) of UBP141 (10 μM). Top traces increpresent averaged superimposed presynaptic SSC action potentials in control and in the presence of UBP141. Right panels: the traces in the absence and in the presence of UBP141 are superimposed. (e) Normalized charge transfer of the train-EPSCs estimated from normalized by amplitude of the first peak currents is increased inTsc1+/−(n=5 cell pairs,N=4 mice) compared withTsc1wtmice (n=7 cell pairs,N=4),P<0.0005, two-tailedt-test. (f) UBP141 decreases the contribution of NMDAR-mediated EPSCs to the postsynaptic summation of EPSCs in synaptically coupled SSCs inTsc1+/−mice. Normalized charge transfer of the train-EPSCs fromTsc1+/−mice in control (n=5 cell pairs,N=4), in the presence (n=4 cell pairs,N=4) and after washout of UBP141 (n=3 cell pairs,N=3).Tsc1+/−versusTsc1+/−in the presence of UBP141,P<0.03, two-tailedt-test). (g) Normalized charge transfer of the train-EPSCs is unaltered in the presence of UBP141 inTsc1wtmice (n=6 cell pairs,P>0.44, two-tailedt-test). All means±s.e.m., *P<0.05, ***P<0.001. NS, not significant. Figure 4: Enhanced temporal integration of synaptic responses in synaptically coupled SSCs in L4 in Tsc1 +/− mice. ( a ) Fluorescence images from two SSCs (left) and the configuration of a paired recordings (right). Scale bar, 50 μm. ( b ) Representative action potential firing patterns of both, postsynaptic (top) and presynaptic (bottom) SSCs recorded in current clamp mode. ( c , d ) Representative averaged normalized by the first peaks in the trains traces of EPSCs recorded in voltage-clamp mode in pairs of SSCs in L4 (averaged 25 sweeps) from Tsc1 wt ( c , bottom panels) and Tsc1 +/− ( d ) mice induced by train stimulation (11 stimuli at 40 Hz) in presynaptic cell in the absence (left panels, black traces) or presence (middle panels, red traces) of UBP141 (10 μM). Top traces in c represent averaged superimposed presynaptic SSC action potentials in control and in the presence of UBP141. Right panels: the traces in the absence and in the presence of UBP141 are superimposed. ( e ) Normalized charge transfer of the train-EPSCs estimated from normalized by amplitude of the first peak currents is increased in Tsc1 +/− ( n =5 cell pairs, N =4 mice) compared with Tsc1 wt mice ( n =7 cell pairs, N =4), P <0.0005, two-tailed t -test. ( f ) UBP141 decreases the contribution of NMDAR-mediated EPSCs to the postsynaptic summation of EPSCs in synaptically coupled SSCs in Tsc1 +/− mice. Normalized charge transfer of the train-EPSCs from Tsc1 +/− mice in control ( n =5 cell pairs, N =4), in the presence ( n =4 cell pairs, N =4) and after washout of UBP141 ( n =3 cell pairs, N =3). Tsc1 +/− versus Tsc1 +/− in the presence of UBP141, P <0.03, two-tailed t -test). ( g ) Normalized charge transfer of the train-EPSCs is unaltered in the presence of UBP141 in Tsc1 wt mice ( n =6 cell pairs, P >0.44, two-tailed t -test). All means±s.e.m., * P <0.05, *** P <0.001. NS, not significant. Full size image GluN2C/D antagonists reduce epileptogenecity in Tsc1 +/− mice The critical role of L4 neurons in increased temporal integration and seizure generation suggests that the selective blockade of long-lasting GluN2C/D subunits containing NMDAR-mediated currents may have antiepileptic effects. To test this possibility, we first used microelectrode array extracellular recordings in acute coronal neocortical slices taken from P15 Tsc1 +/− mice. Spontaneous discharges lasting for up to 10 s were recorded in L2/3 and L4. UBP141 (10 μM) selectively reduced the amount of long-lasting epileptiform episodes, without altering the number of interictal bursts (duration≤500 ms; Supplementary Fig. 10 ). We next tested the antiepileptic actions of UBP141 and DQP1105 in vivo by intraperitoneal (i.p.) injections of the drugs (75 and 28 mg kg − 1 , respectively) to Tsc1 +/− mice. These values were the lowest effective doses identified by testing increasing doses of these compounds (see Methods section for details). In three of six mice tested, the seizures were completely stopped ~40 min after i.p. injection of UBP141, and in the remaining mice ( n =3) there was a seizure-free period lasting 109±39 min ( Fig. 5a,b ). I.p. injection of DQP1105 stopped seizures on average for 72.6±5.5 min in four out of six mice, and seizures were completely stopped in two mice ( Fig. 5c ). In contrast, recurrent epileptic discharges persisted up to 7 h in Tsc1 +/− mice that did not receive the antagonists or were i.p. injected with vehicle ( Fig. 5d,e ). Therefore, selective antagonists of GluN2C/D-containing receptors have in vivo and in vitro antiepileptic actions in Tsc1 +/− mice. 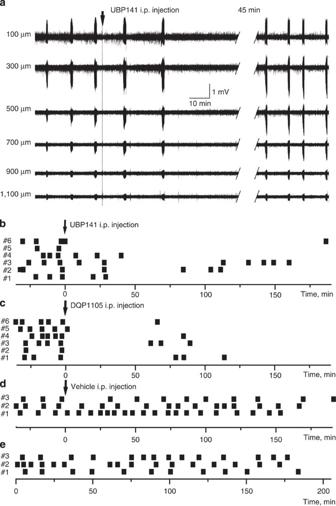Figure 5: Acute antiepileptic effect of i.p. administration of UBP141 or DQP1105in vivo. (a) Intracortical EEG recordings in head-restrained P15Tsc1+/−mouse before and after i.p. administration of UBP141 (75 mg kg−1; indicated by arrow). The upper trace corresponds to the superficial intracortical electrode placed at 100 μM from the pia, channels are separated by 200 μm. (b–e) Time course of spontaneous seizure activity inTsc1+/−mice at P14–P16 before and after i.p. administration of UBP141 (N=6 mice;b), DQP1105 (28 mg kg−1,N=6;c), vehicle control (N=3;d) and control without any treatment (N=3;e). Individual seizures are represented by black squares. Each row (#) represents individual experiment. Figure 5: Acute antiepileptic effect of i.p. administration of UBP141 or DQP1105 in vivo. ( a ) Intracortical EEG recordings in head-restrained P15 Tsc1 +/− mouse before and after i.p. administration of UBP141 (75 mg kg − 1 ; indicated by arrow). The upper trace corresponds to the superficial intracortical electrode placed at 100 μM from the pia, channels are separated by 200 μm. ( b – e ) Time course of spontaneous seizure activity in Tsc1 +/− mice at P14–P16 before and after i.p. administration of UBP141 ( N =6 mice; b ), DQP1105 (28 mg kg − 1 , N =6; c ), vehicle control ( N =3; d ) and control without any treatment ( N =3; e ). Individual seizures are represented by black squares. Each row (#) represents individual experiment. Full size image Importantly, after UBP141 injection a basal activity remained unaltered, in particular, at γ-frequency band ( Supplementary Fig. 11 ), known to be enhanced by common NMDAR antagonists [37] . This might indicate that used dosage of UBP141 corresponds to the concentration in the brain to be within the selectivity range for GluN2C/D. The used dosage of DQP1105 (28 mg kg − 1 ) according to in silico prediction tools appears to be also within the selectivity range for GluN2C/D receptors (see Methods section for details and Supplementary Table 1 ). The direct assessment of the distribution of both drugs in the brain requires further studies. Collectively, our observations on the Tsc1 +/− animal model suggest that seizures are generated intracortically owing to an upregulation of GluN2C receptors in recurrent connections between SSCs in the granular layer of neocortex and then propagate to other layers. Interestingly, in some Tsc1 +/− mice sensory stimulation (mainly back and feet corresponding to receptive field in the recorded cortical zone) induced a seizure ( Supplementary Fig. 12 ), indicating that sensory inputs to L4 may trigger paroxysmal recurrent network activity in the cortex. This strongly reinforces the importance of the hyper-synchronizing effects of L4 and of functional upregulation of GluN2C subunits of NMDARs. GluN2C overexpression in human TSC postsurgical tissue To test whether findings obtained in the animal model can be translated to human patients with TSC, we performed studies in human postsurgical tissue. Quantitative RT–PCR performed in human samples with TSC2 mutation (age at surgery ranged from 8 to 16 months; Supplementary Table 3 ) revealed a 20-fold increase of GluN2C mRNA compared with fetal control brains ( Fig. 6a ; P <0.001, two-tailed t -test) and more than 2.5-fold increase compared with adult control brains. 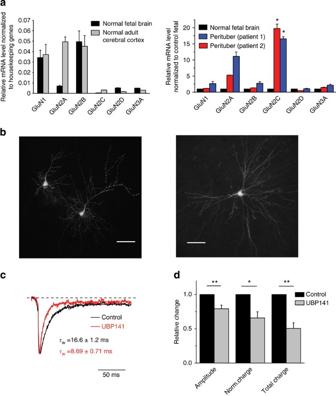Figure 6: Upregulation of GluN2C subunit of NMDARs in human postsurgical tissue of TSC patients. (a) Differential expression of NMDA receptor subunits in human brain tissue from normal individuals and TSC patients. Left panel: quantitative RT-PCR showing the relative expression of mRNAs encoding different NMDAR subunits in normal samples from human fetal (pool of 59 male/female Caucasian fetuses ages 20–33 weeks) and adult (pool of 10 male/female Caucasians ages 20–68 years) cerebral cortex. The error bars indicate ±s.e.m. from two replicates of quantitative RT-PCR experiments for both sets. β-actin and GAPDH were used for normalization. Right panel: fold change expressions for each receptor in two TSC patients calculated relative to the normal fetal brain. The error bars for patient 1 indicate the ±s.e.m. from two replicates of quantitative RT-PCR experiments. The error bars for patient 2 indicate the ±s.e.m. from three samples. All samples were tested in duplicate. (b) Morphology of dysplastic excitatory neurons in cortical slices of human postsurgical tissue of TSC patients. Scale bar, 50 μm applies to both images. (c) Grand averages of normalized (Norm.) and superimposed traces of sEPSC recorded at −50 mV from dysplastic neurons in cortical slices of human postsurgical tissue of three TSC patients in control (pooled data from eight neurons) and in the presence of 10 μM UBP141 (pooled data from seven neurons). (d) Summary data for the effects of 10 μM UBP141 on amplitudes, normalized and total charges of the sEPSC recorded from human postsurgical tissue (relative to corresponding controls,n=7 cells). All means±s.e.m., *P<0.05, **P<0.01; paired two-tailedt-tests. Figure 6: Upregulation of GluN2C subunit of NMDARs in human postsurgical tissue of TSC patients. ( a ) Differential expression of NMDA receptor subunits in human brain tissue from normal individuals and TSC patients. Left panel: quantitative RT-PCR showing the relative expression of mRNAs encoding different NMDAR subunits in normal samples from human fetal (pool of 59 male/female Caucasian fetuses ages 20–33 weeks) and adult (pool of 10 male/female Caucasians ages 20–68 years) cerebral cortex. The error bars indicate ±s.e.m. from two replicates of quantitative RT-PCR experiments for both sets. β-actin and GAPDH were used for normalization. Right panel: fold change expressions for each receptor in two TSC patients calculated relative to the normal fetal brain. The error bars for patient 1 indicate the ±s.e.m. from two replicates of quantitative RT-PCR experiments. The error bars for patient 2 indicate the ±s.e.m. from three samples. All samples were tested in duplicate. ( b ) Morphology of dysplastic excitatory neurons in cortical slices of human postsurgical tissue of TSC patients. Scale bar, 50 μm applies to both images. ( c ) Grand averages of normalized (Norm.) and superimposed traces of sEPSC recorded at −50 mV from dysplastic neurons in cortical slices of human postsurgical tissue of three TSC patients in control (pooled data from eight neurons) and in the presence of 10 μM UBP141 (pooled data from seven neurons). ( d ) Summary data for the effects of 10 μM UBP141 on amplitudes, normalized and total charges of the sEPSC recorded from human postsurgical tissue (relative to corresponding controls, n =7 cells). All means±s.e.m., * P <0.05, ** P <0.01; paired two-tailed t -tests. Full size image Whole-cell patch-clamp recordings in brain slices from the human TSC specimens showed that sEPSCs recorded from dysplastic neurons in granular and supragranular layers ( Fig. 6b ) were significantly reduced and curtailed by UBP141 ( Fig. 6c,d ). The amplitude, total and normalized charges of sEPSC in the presence of UBP141 (10 μM) were 0.78±0.04 ( P <0.002, paired two-tailed t -test, n =7), 0.59±0.08 ( P <0.002, paired two-tailed t -test, n =7) and 0.68±0.09 ( P <0.01, paired two-tailed t -test, n =7), respectively, of controls. The values of τ w of sEPSC decay in TSC samples were 16.6±2.1 ms without UBP141 and 8.69±0.71 ms in the presence of UBP141 ( P <0.0002, two-samples two-tailed t -test, n =7). Furthermore, in two human tissue samples displaying spontaneous paroxysmal activity UBP141 (10 μM) reduced spontaneous spike frequency ( Supplementary Fig. 13 ). Therefore, in conjunction with animal model data functional upregulation of GluN2C may contribute to epilepsy associated with TSC in human patients. Genetic polymorphisms and biochemical markers of mTOR activation have been also identified in patients with isolated focal cortical dysplasia (FCD), a common aetiology of intractable epilepsy [38] , [39] , [40] , [41] , [42] . GluN2B and GluN2C mRNA levels have been found to be upregulated in dysplastic neurons microdissected from human FCD specimens obtained during epilepsy surgery [26] . Therefore, we tested whether slow UBP141-sensitive NMDAR-mediated component is present in dysplastic neurons from patients with FCD. Whole-cell patch-clamp recordings were performed in five human samples (age at surgery ranged from 1 to 14 years; Supplementary Table 4 ). As in the TSC case, sEPSCs recorded from dysplastic neurons in granular and supragranular layers ( Fig. 7a ) were significantly curtailed by UBP141 ( Fig. 7b,c ). The τ w values of sEPSC decay were 22.7±2.9 ms in control ( n =17) and 9.9±0.7 ms in the presence of UBP141 ( n =13, P <0.001, two-sample, two-tailed t -test). The total and normalized charge of sEPSC in the presence of UBP141 (10 μM) were 0.56±0.08 ( P <0.0003, paired t -test, n =12) and 0.59±0.06 ( P <2 × 10 − 5 , paired two-tailed-test, n =12) of controls, respectively. Amplitudes of sEPSC in the presence of antagonists were not significantly different from control: 0.88±0.07 of control ( P >0.16, two-tailed t -test; Fig. 7d ). 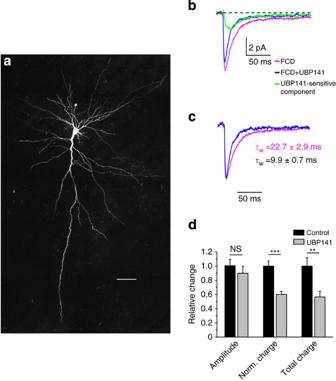Figure 7: Functional upregulation of GluN2C/D subunits of NMDARs in pediatric epilepsy surgery patients with focal cortical dysplasia (FCD). (a) Morphology of dysplastic excitatory neuron in cortical slice of human postsurgical tissue of a patient with FCD. Scale bar, 50 μm. (b) Grand average traces of sEPSC recorded at −50 mV from dysplastic neurons in cortical slices of human postsurgical tissue of five patients with FCD in the absence (red, pooled data from 17 neurons) and in the presence of 10 μM UBP141 (blue, pooled data from 12 neurons). (Green trace)—UBP141-sensitive sEPSC component revealed by subtraction of the trace with UBP141 from the trace without UBP141. (c) Grand average traces of sEPSCs normalized (Norm.) by peak amplitudes. (d) Summary data for the effects of 10 μM UBP141 on amplitudes, normalized and total charges of the sEPSC recorded from human postsurgical tissue relative to corresponding controls. All means±s.e.m., **P<0.01, ***P<0.001.Two-samplet-tests were performed on the pooled data for each parameter (control conditions:n=17 cells, with UBP141:n=12 cells). NS, not significant. Figure 7: Functional upregulation of GluN2C/D subunits of NMDARs in pediatric epilepsy surgery patients with focal cortical dysplasia (FCD). ( a ) Morphology of dysplastic excitatory neuron in cortical slice of human postsurgical tissue of a patient with FCD. Scale bar, 50 μm. ( b ) Grand average traces of sEPSC recorded at −50 mV from dysplastic neurons in cortical slices of human postsurgical tissue of five patients with FCD in the absence (red, pooled data from 17 neurons) and in the presence of 10 μM UBP141 (blue, pooled data from 12 neurons). (Green trace)—UBP141-sensitive sEPSC component revealed by subtraction of the trace with UBP141 from the trace without UBP141. ( c ) Grand average traces of sEPSCs normalized (Norm.) by peak amplitudes. ( d ) Summary data for the effects of 10 μM UBP141 on amplitudes, normalized and total charges of the sEPSC recorded from human postsurgical tissue relative to corresponding controls. All means±s.e.m., ** P <0.01, *** P <0.001.Two-sample t -tests were performed on the pooled data for each parameter (control conditions: n =17 cells, with UBP141: n =12 cells). NS, not significant. Full size image Thus, although our direct results are designed for studying the mechanisms of epileptogenesis associated with TSC1 mutation, they may provide important link for other neurodevelopmental disorders with epilepsy associated with mTOR activation such as FCD. Our observations provide the first evidence that GluN2C NMDARs are functionally upregulated in neurons of heterozygote Tsc1 +/− mice and in human TSC patients. The upregulated expression of GluN2C receptors in neocortical L4 appear as prerequisite for seizure generation in the developing haploinsufficient Tsc1 +/ − mice despite the absence of tubers and are key factors in the mechanisms of intracortical epileptogenesis. In line with this concept, GluN2C/D receptor antagonists stop seizures in vivo and in vitro . Our data with rapamycin-treated mice indicate a crucial role of mTOR signalling in increased functional expression of GluN2C NMDARs in Tsc1 +/− mice. Finally, examination of postsurgical tissue samples from TSC patients revealed that these findings could be potentially translated to human. Overall, our data suggest that GluN2C-subunit targeted therapy provides a promising novel therapeutic avenue to treat epilepsy associated with TSC. Our in vivo recordings show that Tsc1 +/− mice exhibit a variety of seizure types (most often generalized, up to 7 min duration). Fast Fourier transform power spectra analysis of the EEG recordings revealed increased contribution of fast and ultrafast (200–500 Hz) oscillations—an important hallmark of epileptiform activity. EEG patterns in Tsc1 +/− mice resemble those seen in human epileptic seizures, and are typically associated with remarkable behavioural phenotype: freezing, facial automatisms, head tremor, straub tail and tonic-clonic seizures. Seizures in this animal model, therefore, entirely fulfil the criteria and definition of epileptic seizures proposed by the International League Against Epilepsy and the International Bureau for Epilepsy [43] . However, some features and clinical phenotype in this animal model are distinctive from the human disease: in particular in mice seizures spontaneously disappear after P19, whereas in children with TSC seizures are usually highly persistent, although seizure type may change with age. Both Tsc1 and Tsc2 heterozygous knockout mice have been intensively studied in the last years. Tsc1 +/− and Tsc2 +/− mice show social and cognitive deficits in the absence of any apparent major cerebral pathology [4] , [19] , [20] , although loss of a single copy of Tsc gene is sufficient to perturb neuronal morphology, dendritic spine structure [22] and axon guidance [44] . Eventually, it has been proposed as a model in which haploinsufficiency for the Tsc genes leads to aberration in neuronal functioning, including changes in synaptic strength and glutamate receptor composition of excitatory synapses, resulting in impaired learning and social behaviour. Importantly, the mTOR complex 1 (mTORC1) inhibitor rapamycin improves learning and memory deficits in Tsc2 +/− mice [4] , and social deficit in both Tsc1 +/− and Tsc2 +/− mice, suggesting that uncontrolled mTORC1 signalling is a core molecular mechanism involved in the behavioural abnormalities [19] , [45] . Thus, although mice haploinsufficient for the Tsc genes have been utilized as models of autism [4] , [19] , [20] , occurrence of spontaneous seizures in Tsc1 +/− and Tsc2 +/− rodents have not been reported previously [46] . It is possible that early spontaneous epileptic activity in Tsc1 +/− heterozygous knockout mice has been overlooked because of the strictly limited age window (<P19) found in our study. Interestingly, in 82.1% of epileptic TSC patients, the epilepsy begins before 3 years of life [47] . Thus, this early seizure appearance in Tsc1 +/− mice is consistent with the early epilepsy onset in TSC patients. Spontaneous seizure discharges in Tsc1 +/− mice involve neocortical L4 before supra- and infragranular layers, both in vivo and in vitro , indicating layer L4 as a possible origin of seizure generation. L4 is the main acceptor of sensory inputs in which SSCs act as effective integrators of powerful and persistent NMDAR-mediated recurrent excitation [29] , [31] . On the other hand, L4 neurons provide synaptic outputs to virtually all layers in a cortical column (for review, see ref. 27 ). We suggest that in Tsc1 +/− mice, L4 SSCs with functionally upregulated GluN2C receptors become effective ‘hyperintegrators’ of powerful recurrent excitation and intracortical epileptic generator. It has been hypothesized that normal brain circuits provide a template that epileptic brain uses to generate seizures [48] , and in particular that circuits responsible for generating seizure activity are comparable to the circuits that generate spindle bursts [49] . The rhythmic spike-wave discharge has been referred to as a perversion of the spindle oscillation [50] with the circuits within the cortex amplifying the spindle activity. This hypothesis was derived primarily from CSD analysis of cortical region during spindle activity [51] , showing that early significant current sink occurs in cortical L4. This is in line with our own observations. Intriguingly, tactile stimulation of the Tsc1 +/− mouse back induced prominent seizures ( Supplementary Fig. 12 ), indicating that seizure initiation can be triggered by conventional sensory inputs to L4. Extensive recurrent connectivity due to upregulated GluN2C receptors in granular layer provide a source of powerful local excitation and is capable of producing activity that is self-generated and long-lasting. Rhythmic activity in the EEG γ-band is a near-ubiquitous feature of ongoing cortical activity and responses to sensory input, and this activity has been found selectively enhanced in epilepsy [52] . Combined computational and experimental approaches show that high-frequency γ rhythms originate particularly from L4 (ref. 53) [53] . Our data show that slow decay of the GluN2C-mediated current contributes more efficiently to temporal summation at high-frequency activity. Indeed, direct paired recordings of recurrent connections between SSCs in L4 revealed increased temporal integration of excitatory input in Tsc1 +/− mice at γ-band frequency synaptic input. As a result neurons become more depolarized for a longer time window promoting neuronal hypersynchronization within L4. In concordance with patch-clamp data, i.p. injection of GluN2C/D antagonists stopped recurrent seizures in Tsc1 +/− mice in vivo. Intriguingly, the impact of «second-hit» mutation on functional upregulation of slow NMDARs in neurons was negligible. Precisely, controlling the timing and location of Cre expression, we could compare the cell-autonomous effects of loss of Tsc1 in an otherwise unperturbed circuit or loss of both alleles in heterozygous background in contrast to the mouse models where Tsc1 is deleted in all forebrain neurons. The results showed that extent of slow NMDAR receptor contribution was the same irrespectively whether neurons were heterozygote or homozygote for the Tsc1 mutation. This indicates that monoallelic mutation in the Tsc1 gene is sufficient to increase the functional expression of GluN2C receptors. Altered expression NMDAR mRNA has been reported for both human TSC and FCD [24] , [26] . In particular increased levels of GluN2B and GluN2D subunits mRNA were observed in tubers [24] . These data differ from present data where selective upregulation of GluN2C was observed. This discrepancy might be attributed to the difference in methods used and different age group of patients: 1-year-old patients in our study and 4–46-year-old (on average 19.5±6 years) patients in ref. 24 . However, selective upregulation of GluN2C-subunit mRNA in single microdissected dysplastic neurons (shown in ref. 24 ) is in a good agreement with functional upregulation of GluN2C/D subunits shown by our electrophysiological data in individual dysplastic neurons. Importantly, sEPSCs recorded from dysplastic neurons brain slices resected from patients with TSC and FCD were significantly attenuated and curtailed by GluN2C/D antagonists. Thus, given an increased expression of specific NMDAR subunits found in tissue resected from patients with various types of drug-resistant epilepsy [25] , [26] , [54] , [55] , the proposed mechanisms of intracortical epileptogenesis and NMDAR-subunit targeted therapy may be further extended to other types of epilepsy, including FCD, the most frequent congenital lesions causing epilepsy. It should be noted, however, that studies on postsurgery samples from TSC and FCD patients need to be interpreted with some caution. This includes our comparative findings from paediatric tissue from TSC patients (~1-year old) with normal fetal tissue. Non-epileptic normal age-matched control tissue is not available for this human study owing to ethical issues, while comparison with age-matched epileptic tissue with different aetiology may lead to misinterpretation and wrong conclusions. Our results should be replicated in other clinical studies with larger cohorts and rigorous age correlation analysis. The failure of general NMDAR antagonists to treat epilepsy in preclinical studies [56] may result from the need to restrict the NMDARs blockade to the specific subunits involved in epileptogenesis in TSC leaving intact pro-survival GluN2A-mediated signalling involved in normal development, plasticity, learning and memory [57] . Administration of non-specific NMDAR antagonists alters γ rhythms and can induce cognitive as well as psychosis-like symptoms in humans [58] . In FS parvalbumin-positive interneurons, NMDARs have a critical role for expression of normal γ rhythms and specific cognitive behaviours [59] . The disruption of NMDAR signalling specifically in parvalbumin-positive interneurons may lead to neural network dysfunction that could underlie these symptoms. The NMDARs present in FS interneurons, both in Tsc1 wt and Tsc1 +/− mice, were not affected by selective GluN2B or GluN2C/D antagonists in our experiments. This suggests that treatment with these compounds does not alter inhibition provided by FS interneurons. Furthermore, power of γ oscillations of basal activity recorded in Tsc1 +/− mice in vivo was not affected by UBP141. Abnormal signalling in the mTOR pathway is known to be critical for the pathophysiology of epilepsy and other neurological features of TSC, and other focal cortical malformations. In animal models of TSC and cortical dysplasia, hyperactivation of the mTOR pathway promotes epileptogenesis and neuropathological abnormalities, and the mTOR inhibitor, rapamycin, prevents epilepsy and associated cellular and molecular phenotypes [2] , [3] , [4] , [60] . Altered mTOR pathway signalling was found in TSC, FCD, hemimegalencephaly and ganglioglioma brain tissue specimens [38] , [40] , [61] , [62] , [63] . The term ‘TORopathies’ was recently coined to define a continuum of neurological disorders characterized by altered cortical architecture, abnormal neuronal morphology and intractable seizures as a consequence of abnormal mTOR signalling [63] , [64] . There is strong evidence supporting a role for mTORC1 in regulating the translation of a number of proteins necessary for synaptic plasticity [65] , and there is a possibility that mTORC1 also regulates translation of GluN2C. Our findings obtained from TSC animal model may, therefore, also have implications for other conditions in which mTORC1 is hyperactive, ranging from Fragile X syndrome to autism spectrum disorders [66] . Animals Breeding and experimental procedures were carried out in accordance with European guidelines for animal research and in accordance with Institut National de la Santé et de la Recherche Medicale guidelines for animal care in research, and were approved by the local ethics committee (Comité d’éthique en expérimentation animale de Marseille (C2EA-14)). Heterozygote Tsc1 wt/mut ( Tsc1 +/− , National Cancer Institute (NCI, USA)) male mice were kindly provided by Dr A. Bordey (Yale University, USA), and Tsc1 flx/flx were obtained from Jackson Laboratories. The genetic background of Tsc1 wt/mut mice was B6;129S4 and Tsc1 flx/flx mice were from a mixed background (C57BL/6J, BALB/cJ, or 129/SvJae mice). These lines of mice were generated by David J. Kwiatkowski (Brigham and Women’s Hospital, Harvard Medical School, Cambridge, MA, USA). Inbred C57BL/6J wild-type ( Tsc1 +/+ ) females were from Janvier Labs (France). Mice were housed in ventilated, light-tight, sound-isolated chambers under standard 12:12 light/dark cycle (light on at 07.00 PM and light off at 07.00 AM) with food and water available ad libitum . Genotyping of pups issued from breading of C57BL/6J Tsc1 +/− males and C57BL/6J Tsc1 +/+ females mice was performed on tail tissue samples at postnatal days P11–P12. The study was conducted in Tsc1 +/− and Tsc1 +/+ mice of both sexes issued from the same litters at P9–P33. In utero electroporation Timed pregnant female mice at the E16 (E0 is counted as the morning on which the vaginal plug is detected) were anaesthetized with a mixture of ketamine (10 mg kg − 1 )/xylazine (100 mg kg − 1 ). The uterine horns were exposed, and a lateral ventricle of each embryo was injected using pulled glass capillaries and a microinjector (Picospritzer II; General Valve) with Fast Green (2 mg ml − 1 ; Sigma, USA) combined with the following DNA constructs: 0.5 mg ml − 1 pCAG-mRFP either alone or with 1.5 mg ml − 1 pCAG-Cre:GFP. Plasmids were further electroporated by discharging a 4,000-mF capacitor charged to 35 V with a BTX ECM 830 electroporator (BTX Harvard Apparatus). The voltage was discharged in five electrical pulses at 950-ms intervals via 5-mm electrodes placed on the head of the embryo across the uterine wall. Quantitative RT–PCR Total RNA was isolated from mouse cerebral cortex and human brain tissue using RNeasy-Plus Mini Kit according to the manufacturer’s protocol (Qiagen). cDNA was synthesized using the Quantitect Reverse Transcription Kit, according to the manufacturer’s protocol (Qiagen). Quantitative real-time RT-PCR experiments were performed using oligonucleotides specific for mouse hypoxanthine phosphoribosyltransferase 1 and cyclophilin-A; human β-actin and GAPDH, and mouse and human NMDAR subunits genes (oligonucleotide sequences are shown in Supplementary Table 5 ). Amplification was done using SYBR-Green and Chemistry (Roche Diagnostics) and Roche amplification technology (Light Cycler 480). All experiments were performed in duplicate or triplicate. To avoid any bias, all samples were blinded before analysis. Only after the final samples were analysed and described, the samples were genotyped. Human fetal brain and adult cerebral cortex mRNAs, used as controls, were purchased from BD Biosciences Clontech (Palo Alto, CA, USA). Animal slice preparation Tsc1 +/+ and Tsc1 +/− mice (P14–P16) were anaesthetized with ether and killed by decapitation in agreement with the European Directive 86/609/EEC requirements. The brain was rapidly removed and placed in an oxygenated ice-cold saline buffer. Transverse 300-μm-thick coronal slices were cut using a vibratome (Leica VT1000S; Leica Microsystems Inc., Deerfield, IL, USA) in ice-cold protecting solution oxygenated with 95% O 2 and 5% of CO 2 . Before recording, slices were incubated in an artificial cerebrospinal fluid (ACSF-1) solution containing (in mM): 125 NaCl, 3.5 KCl, 1 CaCl 2 , 2 MgCl 2 , 1.25 NaH 2 PO 4 , 26 NaHCO 3 and 10 glucose, equilibrated at pH 7.3 with 95% O 2 and 5% CO 2 at room temperature (22–25 °C) for at least 1 h to allow recovery. For the recordings, we used ACSF of the same composition but with 2 mM of CaCl 2 and 1 mM of MgCl 2 (ASCF-2). Immunostaining procedures For immunostaining, P14–P16 mouse brains were perfused with Anti-genfix solution and sliced at 100 μm on a vibratome (Microm). Slices were blocked at room temperature for 1 h with 5% normal goat serum (NGS) and 0.3% Triton X-100 in phosphate-buffered saline (PBS) and incubated overnight at 37 °C with the upper cortical layer marker CDP/CUX1 (M-222 Santa Cruz Biotechnology; 1/200). Human cortical slice preparation After surgical resection, the cortical tissue was placed within 30 s in ice-cold oxygenated protecting solution that contained in (mM): 110 choline chloride, 26 NaHCO 3 , 10 D -glucose, 11.6 sodium ascorbate, 7 MgCl 2 , 3.1 sodium pyruvate, 2.5 KCl, 1.25 NaH 2 PO 4 and 0.5 CaCl 2 , 300 mOsm and transported to the neurophysiology laboratory, within <5 min. Cortical slices (400–900 μm) were prepared in the same solution, and were then transferred to holding chambers in which they were stored at room temperature (20–22 °C) in ACSF-1. Recordings were performed in ACSF-2. Electrophysiological recordings from brain slices Slices were transferred to the recording chamber and perfused with oxygenated recording ACSF-2 at 3 ml min − 1 . Neurons were visualized using infrared differential interference contrast microscopy. Whole-cell patch-clamp recordings were performed at room temperature by using either an EPC-9 amplifier and Patch Master software (HEKA Elektronik, Germany) or Multiclamp 700B amplifier (Molecular Devices, Sunnyvale, CA, USA) and custom-made software based on IgorPro and filtered at 3–10 kHz. Patch pipettes were pulled from borosilicate glass capillaries (World Precision Instruments, Sarasota, USA) and had resistances of 4–6.5 MΩ when filled with the internal solution of the following composition (in mM): 130 K-gluconate, 10 Na-gluconate, 4 NaCl, 4 MgATP, 4 phosphocreatine, 10 HEPES and 0.3 GTP (pH 7.3 with KOH). Biocytin (final concentration 0.3–0.5%) was added to the pipette solution to label the neurons from which recordings were obtained. The series resistance estimated from the amplitude of the initial capacitive transient in response to a 5-mV pulse was 8–24 MΩ. It was not compensated and was monitored during each experiment. Experiments were terminated if the series resistance changed by >15%. Spontaneous EPSCs were recorded for 15 min at −80 mV (the reversal potential for GABAergic currents) and at −50 mV (potential at which the block of NMDAR by magnesium is largely relieved). All recordings were made in ACSF-2 without any proepileptic pharmacological drug. To minimize potential sampling bias, the pups from at least three deliveries for each condition were studied. Analysis and statistics of in vitro data The Mini Analysis 6.0.3 software (Synaptosoft Inc., Decatur, GA, USA) was used to analyse the parameters of synaptic events. The threshold amplitude for detecting EPSCs was set at twice the baseline noise (root mean square), and the EPSCs detected by the software were visually inspected to minimize errors. Events that did not show a typical synaptic waveform were rejected manually. For analysis, only events that did not show any signs of multiple peaks (that is, contamination of rise or decay phases by subsequent events) were selected for subsequent analysis of the kinetics and for exponential fitting. Averaged traces of sEPSC or mEPSC and cumulative probabilities of amplitude and frequency for all cells were obtained using (Mini Analysis; Synaptosoft) software and further analysed with Origin software (MicroCal, Northampton, MA, USA). For each neuron, original traces from individual experiments were aligned based on the starts of their rising phases and averaged. These averaged traces from individual experiments were averaged to form grand average traces. To quantify the current decay kinetics, we measured charge transfer of sEPSC normalized by the peak amplitude. A larger charge transfer corresponds to slower decay kinetics and vice versa. Normalized charge transfer was calculated by the integrating the area under the current waveform in the interval of time between peak of sEPSC and 300 ms after the peak for each individual cell ( Supplementary Fig. 14 ). In addition, to compare decay times between genotypes weighted time constant of sEPSC or mEPSC decay ( τ w ) were calculated using the formula (equation 1): where I is the amplitude of the fast or slow component, and τ is the respective decay time constant. Data are expressed as mean±s.e.m. All comparisons were two-tailed t -tests or one-way ANOVA with post hoc Fisher’s Least Significant Difference multiple comparison. Statistical significance for cumulative probabilities was estimated using Kolmogorov–Smirnov and Mann–Whitney tests. From three to nine animals were used for each data set. Immunocytochemistry After the recording session, to visualize and identify the recorded neurons, we visualized the biocytin injected during whole-cell recordings. After 24 h in paraformaldehyde (3%) at 4 °C, the sections were rinsed in PBS and pre-incubated for 1 h in 0.3% Triton X-100 (Abcys) in PBS with 5% NGS at room temperature. Slices were then incubated in Streptavidin-Cy3 (1:500) in PBS Triton X-100 (0.3%) and NGS (5%) during 12 h at 4 °C. After thorough rinsing, slices were mounted in fluoromount and coverslipped. In vivo recordings and data analysis Experiments were performed on postnatal days P9–P33 of inbred C57BL/6J strain of both sexes of Tsc1 +/− and Tsc1 wt mice from the same litters issued from breading of Tsc1 wt females and Tsc1 +/− males. The available littermates mice were randomly picked out of the cage and genotyped after experiments. Surgery was performed under isoflurane anaesthesia. In brief, the skull of the animal was cleaned of skin and periosteum. The skull was covered by glue and dental cement except for a 4–9 mm 2 window above the somatosensory cortex from one or two hemispheres. Two plastic bars were fixed to the nasal and occipital bones of the pups head by dental cement. After surgery, animals were warmed and were left for an hour for recovery from anaesthesia. During recordings, the head was fixed to the frame of the stereotaxic apparatus by attached bars; animals were surrounded by a cotton nest and heated via a thermal pad (36.6–37.7 °C). A silver chloride reference electrode was placed in the cerebellum or visual cortex. EEG recordings were performed in non-anaesthetized head-restrained Tsc1 +/− and control Tsc1 wt mice. Sixteen site-linear silicon probe (100 μm separation distance between recording sites, Neuronexus Technologies, MI, USA) was placed into the somatosensory cortex using the Paxinos and Franklin atlas (2001) at coordinates: anterior–posterior=2–2.5 mm, mediolateral=2–3 mm from Bregma, 1.2–1.5 mm depth, to trace the columnar activity at all layers and CA1 zone of the hippocampus. Signals were amplified ( × 100) and filtered at 3 kHz using a 16-channel amplifier (A-M systems, Inc.), digitized at 10 kHz and saved to hard disk of PC using Axoscope software (Molecular Devices). Recordings were analysed offline using Clampfit and MATLAB software (The Mathworks, Natick, MA, USA). After the recordings, position of silicone probe was verified visually by DiI staining of the electrode in 100 μm coronal sections from fixed brain. The actions of UBP141 and DQP1105 were studied in vivo animal model of TSC in keeping with recent guidelines for preclinical candidate drug evaluation [67] . We considered that multiunit activity occurred in epileptic discharges if they appeared in a group of multiple spikes whose amplitude exceeded at least twice the background activity within a period lasting for at least 20 s. The first and last spikes of each discharge were used to define its onset and termination, respectively. For each discharge, amplitude was defined as the amplitude of the largest spike of the discharge. During EEG recordings, animals were monitored visually to determine behavioural correlates of each electrographic epileptic discharge. For EEG data analysis, raw data were preprocessed using a custom-developed suite of programs in the MATLAB analysis environment. The wide-band signal was downsampled to 1,000 Hz and used for local field potential (LFP) signal. Positive polarity is graphed as up throughout the whole manuscript. LFPs were analysed by custom-written, MATLAB-based programs. Approximate anatomical location of each recording site was estimated by physical depth within the brain and corresponding age-matched histological assessment of respective layers depth. Negative epileptic events were detected by the following steps: (1) the LFP signal was band-pass filtered (5–100 Hz); (2) the times of negative troughs with amplitude >5 s.d. from baseline level were detected from filtered signal; and (3) aligned by the times of detected negative epileptic events; the LFP segments from all channels were taken. Note that the length of the segment is 200 ms with moment of negative trough at 0. CSD analysis across cortical depth was used to eliminate volume conduction and localize synaptic currents. CSD was computed for each recording site according to differential scheme for second derivative and smoothed with a triangular kernel of length 3. Preliminary screen for UBP141 and DQP1105 efficacy in vivo Saline solution (200 μl), UBP141 (200 μl, 75 mg kg − 1 ) and DQP1105 (200 μl, 28 mg kg − 1 ) were injected i.p. Using in silico prediction of blood–brain barrier permeation, we estimated expected concentration of compounds in the brain. The decimal logarithm of brain to blood concentration ratio (logBB) and drug concentration relationship in the brain and blood (plasma) tissues were reconstructed using the Clark’s equation [68] to assess the logBB value for the UBP141 and DQP1105 compounds (equation (2)): where ClogP is a calculated octanol-water partitioning coefficient, and PSA is a polar surface area ( Supplementary Table 6 and Supplementary Fig. 15 ). Both parameters were determined from molecular fields using the VolSurf+ molecular modelling software programme (Molecular Discovery Ltd, Perugia, Italy) [69] . According to this model the pharmacodynamic distribution of the drugs in the brain after i.p. injection was assessed at least as 6.7% and 15% of the initial concentration in blood for UBP141 and DQP1105, respectively. On the other hand, according to ref. 70 , the free-drug concentration in the peritoneal cavity is described as its exponential decrease over distance ( x ) from the serosal surface (peritoneum) since the drug diffuses down the concentration gradient into the bloodstream ( Supplementary Fig. 16 ). At characteristic diffusion length, × 0 (average distance travelled by drug molecules), the concentration difference between tissue and blood is decreased to 37% of its maximum value. Therefore, considering the decline of drug concentration at × 0 due to peritoneal transport, and the logBB values the distribution of DQP1105 in the brain after i.p. injection can be assessed. Assuming DQP1105 concentration in injected solution (2.5 mM), volume of injection (200 μl) and total circulating blood volume (of ~1,000 μl), concentration in brain will be around 25 μM that is entirely within the selectivity range for GluN2C/D ( Supplementary Table 1 ). Similar estimation for UBP141 is complicated by the fact that effect of UBP141 (in contrast to DQP1105) was delayed for 40 min after i.p. injection, and unknown pharmacokinetic profile could significantly influence the estimation. Preliminary screen for efficacy of UBP141 and DQP1105 was also performed directly to detect threshold for antiepileptic activity. In 12 animals tested, i.p. injection of UBP141 with dosages of 19 or 57 mg kg − 1 did not produce significant antiepileptic effects. In three animals tested, i.p. injection of DQP1105 with a dosage of 14 mg kg − 1 was also ineffective. A dosage of 75 mg kg − 1 for UBP141 and 28 mg kg − 1 for DQP1105 were the lowest effective doses identified by testing increasing doses of these compounds. Multisite extracellular recordings from brain slices Multisite extracellular recordings of spontaneous activity in slices were performed at 30–32 °C using Multi-electrode array (MEA) made up of 60 planar microelectrodes (TiN/SiN, 30 μm electrode diameter, 200 μm pitch) arranged over an 8 × 8 square grid (Multi Channel Systems (MCS), Reutlingen, Germany). Slices were maintained in dishes and perfused with oxygenated recording ACSF-2. The spontaneous activity was monitored and recorded for 30–120 min, starting 15–20 min after setting slice in the recording chamber at a stable level of activity. After 1,200 × amplification (MCS MEA 1060), signals were sampled at 10 kHz using the MCS data acquisition card controlled by the MCS MCRack software. Data were analysed offline by using custom software tools specifically developed in MATLAB . Chemicals All drugs were prepared as concentrated stock solutions (10–100 mM), stored frozen and then thawed and diluted in ACSF-2 immediately before use. Ro-25697 (αR,βS)-α-(4-hydroxyphenyl)-β-methyl-4-(phenylmethyl)-1-piperidinepropanol maleate, and DQP1105 5-(4-bromophenyl)-3-(1,2-dihydro-6-methyl-2-oxo-4-phenyl-3-quinolinyl)-4,5-dihydro-g-oxo-1H-pyrazole-1-butanoic acid were purchased from Tocris Biosciences (Bristol, UK). UBP 141 (2R*,3S*)-1-(phenanthrenyl-3-carbonyl)piperazine-2,3-dicarboxylic acid was purchased from Abcam Biochemicals (UK). All other chemicals used for electrophysiology were from Sigma. Treatment with rapamycin Rapamycin (ready-made solution, Sigma-Aldrich, USA, 2.5 mg ml − 1 in DMSO (2.74 mM)) was diluted with saline to a final concentration 0.125 mg ml −1 immediately before use. The mice received single dose of rapamycin (3 mg kg −1 ) by i.p. injection (100 μl) or were injected by the equal volume of vehicle once daily for 8 consecutive days. The electrophysiological recordings were performed 24 h after the last administration. Human subjects Cortical tissue samples were obtained from three TSC epilepsy patients undergoing surgery at the Departments of Pediatric Neurosurgery of Rothschild Foundation (Paris) and Hopital La Timone (Marseille). Informed consent for the use of postsurgical tissue for research purposes was obtained with protocols approved by the Rothschild Foundation and Hopital La Timone review boards. Personal data are stored into a specific database, which is declared to the La Commission nationale de l'informatique et des libertés (CNIL). Bioethical declaration procedure, related to conservation and preparation of human body elements for scientific aims, was achieved during 2011 as referred to the ‘Collection NeurochirEpilepsie‘ under file number DC-2011-1378, and has been approved by Le Comite de Protection des Personnes Ile de France II and Ministère de l'enseignement supérieur et de la recherche. The main clinical and neuropathological characteristics of the study population are summarized in Supplementary Tables 3 and 4 . TSC and FCD specimens were collected from patients who underwent surgery for medically intractable epilepsy. All patients were clinically diagnosed with TSC and FCD and presented a history of epilepsy. How to cite this article: Lozovaya, N. et al. Selective suppression of excessive GluN2C expression rescues early epilepsy in a tuberous sclerosis murine model. Nat. Commun. 5:4563 doi: 10.1038/ncomms5563 (2014).